Graphene-based wireless bacteria detection on tooth enamel Direct interfacing of nanosensors onto biomaterials could impact health quality monitoring and adaptive threat detection. Graphene is capable of highly sensitive analyte detection due to its nanoscale nature. Here we show that graphene can be printed onto water-soluble silk. This in turn permits intimate biotransfer of graphene nanosensors onto biomaterials, including tooth enamel. The result is a fully biointerfaced sensing platform, which can be tuned to detect target analytes. For example, via self-assembly of antimicrobial peptides onto graphene, we show bioselective detection of bacteria at single-cell levels. Incorporation of a resonant coil eliminates the need for onboard power and external connections. Combining these elements yields two-tiered interfacing of peptide–graphene nanosensors with biomaterials. In particular, we demonstrate integration onto a tooth for remote monitoring of respiration and bacteria detection in saliva. Overall, this strategy of interfacing graphene nanosensors with biomaterials represents a versatile approach for ubiquitous detection of biochemical targets. Interfacing electronic devices and sensors with biomaterials has been of interest for decades, for on-body physiological and analytical measurements [1] , [2] , [3] . Traditionally, device designs for such applications involved either implantation of device electrodes into tissue [4] , or mechanical mounting of components on the body using braces, clamps or adhesive tapes. Such systems encased rigid and bulky onboard power sources, associated circuitry, and direct physical connections between the sensing probes and data processing electronics [5] , [6] . Further, the large form factors and rigid substrates prohibited intimate integration on the soft and curvilinear surfaces of biological tissues, causing discomfort during continuous use. Device designs and platforms that minimize the mechanical discrepancy between such abiotic/biotic interfaces are thus highly desired for conformal biointegrated electronics and sensors. Electronic sensors based on nanoscale materials such as nanowires [7] , carbon nanotubes (CNTs) [8] and graphene [9] have been shown to boast parts-per-billion sensitivities, a consequence of the high surface areas of these materials. CNT-based composite materials with passive circuits have enabled wireless chemical and gas sensors [10] . Single-atom-thick, sp 2 graphene is a particularly interesting material owing to its remarkable electrical [11] , mechanical [12] and sensing [13] , [14] properties. The growth of graphene films on supporting metallic films (Ni or Cu) using chemical vapour deposition methods [15] , combined with post-etching of the underlying metal, offers the ability to efficiently transfer graphene films to other substrates over large areas [16] for biocompatible sensing and flexible electronics applications [17] , [18] . This is enabled by graphene's intrinsic strength of 42 N m −1 and Young's modulus of ∼ 1 TPa [19] , as well as the high interfacial adhesion exhibited by graphene to substrates (adhesive energy of 0.45 J m −2 on SiO 2 ) [20] . These properties render graphene an ideal active material for direct interfacing onto rugged surfaces. Silk, a textile industry staple for thousands of years, has recently sparked increased interest within the materials science community owing to its impressive mechanical properties, including high elastic modulus, tensile strength, ductility and toughness [21] , [22] . As a result, silk films have been shown to be an efficient 'middleman' medium for transferring materials such as passive metallic electrodes onto tissues via intimate contact and dissolution. This is a consequence of the elasticity and biodegradability imparted by the unique molecular structure of silk. Silk films have been patterned with metal electrodes and intimately 'bioresorbed' onto brain and skin tissues for electro-mapping experiments [21] , [23] . Recent work has demonstrated the ability to fabricate active electronic components such as transistors [24] and metamaterials [25] on films of regenerated silk. In addition to sensor sensitivity, selectivity towards defined chemical and biological targets is a challenging goal in which bioinspired approaches are particularly useful. Aptamer-functionalized nanotube electrodes have been shown to detect single bacterial cells in real time [26] . Further, we have recently shown that phage display can be utilized to determine peptide sequences that selectively bind to CNTs and graphene [8] , [27] , [28] , [29] . This has enabled the generation of bifunctional peptides containing a carbon nanomaterial recognition moiety combined with an analyte binder to non-covalently self-assemble and impart selectivity on graphene sensor arrays. Another recent study has demonstrated the ability of naturally occurring antimicrobial peptides (AMPs) to serve as robust biorecogniton moieties in electronic biosensing platforms [30] . Unlike antibodies, AMPs are significantly more stable and exhibit broadband detection for a range of pathogenic bacteria [31] , [32] . Pathogenic contamination and resistant 'superbug' infections remain critical concerns in both developed and developing nations, due to extremely low minimum infective doses (MID) for many bacteria and the lack of inexpensive and portable methods to detect at these limits [33] . Currently available methods for the detection of microbiological threats utilize specific enrichment media to separate, identify and count bacterial cells [26] . Alternatively, PCR [34] and DNA-based nanobarcode [35] detection strategies have proven to be fast and highly sensitive, but such methods require pretreatment and cell lysis to extract DNA. An alternative strategy is the development of methods that allow for direct and sensitive detection of whole microbial cells or endotoxins. Particularly interesting would be sensors that could be directly interfaced with contamination sources, including the body, food and hospital equipment. Here, we describe a novel approach to interfacing passive, wireless graphene nanosensors onto biomaterials via silk bioresorption. First, graphene nanosensors are comprehensively printed onto water-soluble silk thin-film substrates. The graphene is then contacted by interdigitated electrodes, which are simultaneously patterned with an inductive coil antenna. Finally, the graphene/electrode/silk hybrid structure is transferred to biomaterials such as tooth enamel or tissue, followed by functionalization with bifunctional graphene–AMP biorecognition moeities. The resulting device architecture is capable of extremely sensitive chemical and biological sensing, with detection limits down to a single bacterium, while also wirelessly achieving remote powering and readout. The generation of 'biotransferrable' sensors combined with high sensitivity and selectivity may provide a first line of defence against pathogenic threats at the point of contamination. Graphene/silk sensor The fundamental operation and key functionalities of the sensor design are schematically illustrated in Fig. 1 . First, a graphene-based sensing element with wireless readout coil is generated on silk fibroin ( Fig. 1a ). Next, the ultra-thin nanosensors are intimately biotransferred from the silk platform onto biomaterials, such as tooth enamel, via dissolution of the supporting silk film ( Fig. 1b ). The extremely large surface area of the graphene and electrodes ensures high adhesive conformability to the rugged surfaces of biomaterials. Specificity in biological recognition is achieved by self-assembling designer bifunctional AMP-graphene peptides onto the graphene monolayer ( Fig. 1c ), so graphene functionalization can be achieved without degrading its electronic sensing properties. Further, Fig. 1c illustrates the two other major functionalities of the hybrid biosensor unit: battery-free operation and remote wireless sensing capability. Upon recognition and binding of specific bacterial targets by the immobilized peptides ( Fig. 1d ), the electrical conductivity of the graphene film is modulated and wirelessly monitored using an inductively coupled radio frequency (RF) reader device. The key functionalities of the graphene/silk hybrid sensing elements are thus derived from a synergistic integration of the individual materials properties and components. 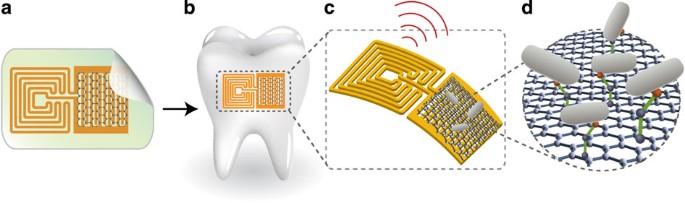Figure 1: Biotransferrable graphene wireless nanosensor. (a) Graphene is printed onto bioresorbable silk and contacts are formed containing a wireless coil. (b) Biotransfer of the nanosensing architecture onto the surface of a tooth. (c) Magnified schematic of the sensing element, illustrating wireless readout. (d) Binding of pathogenic bacteria by peptides self-assembled on the graphene nanotransducer. Figure 1: Biotransferrable graphene wireless nanosensor. ( a ) Graphene is printed onto bioresorbable silk and contacts are formed containing a wireless coil. ( b ) Biotransfer of the nanosensing architecture onto the surface of a tooth. ( c ) Magnified schematic of the sensing element, illustrating wireless readout. ( d ) Binding of pathogenic bacteria by peptides self-assembled on the graphene nanotransducer. Full size image Materials integration and characterization Large-area graphene monolayers are integrated with water-soluble silk fibroin films (ca. 50 μm thick) using a simple transfer printing process ( Fig. 2a , see Methods). Electrode patterns are then incorporated onto the silk–graphene hybrid films via shadow mask-assisted electron beam evaporation of gold to generate the biosensor ( Fig. 2b ). Specifically, the architecture consists of a parallel LRC resonant circuit with a gold inductive coil for wireless transmission, and interdigitated capacitive electrodes contacting graphene resistive sensors. The resulting device is a passive wireless telemetry system, obviating onboard power sources and external connections. A full-wave electromagnetic simulation tool, Ansoft HFSS, was utilized to simulate and design the planar coil antenna and interdigitated capacitive electrode geometries (Methods and Supplementary Fig. S1 ). 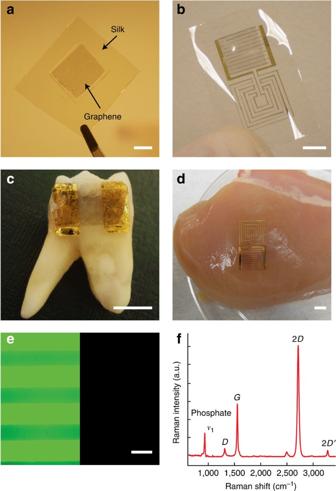Figure 2: Graphene biotransfer and characterization. (a) Graphene printed onto bioresorbable silk film. (b) Passive wireless telemetry system consisting of a planar meander line inductor and interdigitated capacitive electrodes integrated onto the graphene/silk film. (c,d) Graphene nanosensor biotransferred onto the surface of a human molar (c) and onto muscle tissue (d). Scale bars are 5 mm. (e) Fluorescent image of the sensor fabricated on a fluorescent silk film and laminated onto the surface of a tooth, before (left) and after (right) dissolution of silk. Absence of fluorescence signal confirmed complete removal of the silk matrix. Scale bar is 250 μm. (f) Raman spectrum following interfacing of graphene onto the tooth surface. Figure 2: Graphene biotransfer and characterization. ( a ) Graphene printed onto bioresorbable silk film. ( b ) Passive wireless telemetry system consisting of a planar meander line inductor and interdigitated capacitive electrodes integrated onto the graphene/silk film. ( c , d ) Graphene nanosensor biotransferred onto the surface of a human molar ( c ) and onto muscle tissue ( d ). Scale bars are 5 mm. ( e ) Fluorescent image of the sensor fabricated on a fluorescent silk film and laminated onto the surface of a tooth, before (left) and after (right) dissolution of silk. Absence of fluorescence signal confirmed complete removal of the silk matrix. Scale bar is 250 μm. ( f ) Raman spectrum following interfacing of graphene onto the tooth surface. Full size image The thin-film sensing elements thus fabricated on silk are then biotransferred and intimately integrated onto a variety of substrates. Complete dissolution of the silk matrix template in water led to a strong attachment of the graphene–Au electrode structure within a time period of 15–20 min. Significantly, Fig. 2c shows a photograph of the graphene nanomaterial with patterned gold electrodes biointerfaced onto the surface of a human molar, and Fig. 2d shows a photograph of the graphene sensor biotransferred directly on muscle tissue (integration on human skin is shown in Supplementary Fig. S2 ). Optical characterization of the transferred graphene revealed good structural integrity ( Supplementary Fig. S3 ; for sensors interfaced with skin, no degradation or delamination was observed following mild rinsing in running water as shown in Supplementary Fig. S4 ). To ensure complete dissolution of the silk substrate, we performed sensor biotransfer experiments using fluorescent silk films, before and after the dissolution of the silk ( Fig. 2e , left). Complete quenching of fluorescence was verified after immersion in water for 20 min ( Fig. 2e , right). Electronic and structural properties of the graphene were interrogated using Raman spectroscopy [36] : Fig. 2f shows the Raman spectrum of graphene following biotransfer onto a tooth surface (Raman spectra of the bare tooth enamel and silk fibroin film are provided in Supplementary Fig. S5 ). The spectrum is in good agreement with other graphene monolayer spectra [36] , and the phosphate ν 1 peak from the tooth enamel substrate is evident [37] . The mechanical stability of the sensor on tooth enamel was analysed via agitation in commercial mouthwash for a period of 3 min followed by comparative Raman spectra analysis ( Supplementary Fig. S6 ). Functionalization of graphene with AMPs The ability to specifically detect various species of pathogenic bacteria is useful for biomedical applications, and food, water and air quality monitoring. Our previous study [30] demonstrated that AMPs may serve as robust biorecognition molecules with broad-spectrum activity towards various pathogenic bacteria. Further, we have recently shown that phage display can be utilized to determine peptide sequences, which selectively bind to carbon nanomaterials [8] , [27] , [38] . Here, graphene nanosensors were functionalized with a chemically synthesized bifunctional peptide, consisting of a dodecapeptide graphene-binding peptide (GBP), a triglycine linker and the AMP odorranin-HP (OHP), which shows activity towards both the Gram-negative bacteria Escherichia coli and Helicobacter pylori , and the Gram-positive bacteria Staphylococcus aureus [39] . 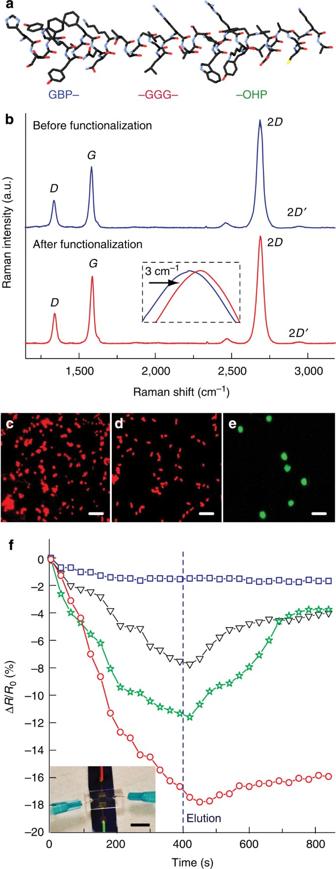Figure 3: Graphene functionalization with AMPs. (a) Molecular model of a bifunctional peptide consisting of a GBP coupled to an AMP OHP via a triglycine linker (–GGG–). (b) Raman spectra before (blue line) and after (red line) immobilization of bifunctional peptides on the graphene surface. The inset shows a shift in the 2Dband of graphene due to molecular doping. (c–e) Fluorescent images of the binding ofS. aureus(c),H. pylori(d) and erythrocytes (e) to GBP–OHP-functionalized graphene. Scale bars are 10 μm. (f) Selectivity of GBP–OHP-functionalized graphene sensor. Blue squares indicate resistance of graphene sensor functionalized with GBP–OHP upon exposure to DI water. Black triangles indicate resistance of graphene sensor functionalized with only GBP upon exposure toS. aureus. Green stars indicate resistance of graphene sensor functionalized with GBP–OHP upon exposure to erythrocytes. Red circles indicate resistance of graphene sensor functionalized with GBP–OHP upon exposure toS. aureus. Dotted line indicates elution with DI water. Inset shows image of the flow-through measurement system. Scale bar is 1 cm. Concentration of the bacterial cells used for the assays is 106CFU ml−1, and the concentration of erythrocytes is 40% haematocrit. Figure 3a shows a molecular drawing of the resulting 38 amino-acid sequence, HSSYWYAFNNKT-GGG-GLLRASSVWGRKYYVDLAGCAKA (GBP–OHP). Raman spectroscopic analysis of the peptide-functionalized graphene surface indicated slight doping of graphene ( Fig. 3b ), consistent with our previous electronic measurements [38] . Figure 3: Graphene functionalization with AMPs. ( a ) Molecular model of a bifunctional peptide consisting of a GBP coupled to an AMP OHP via a triglycine linker (–GGG–). ( b ) Raman spectra before (blue line) and after (red line) immobilization of bifunctional peptides on the graphene surface. The inset shows a shift in the 2 D band of graphene due to molecular doping. ( c – e ) Fluorescent images of the binding of S. aureus ( c ), H. pylori ( d ) and erythrocytes ( e ) to GBP–OHP-functionalized graphene. Scale bars are 10 μm. ( f ) Selectivity of GBP–OHP-functionalized graphene sensor. Blue squares indicate resistance of graphene sensor functionalized with GBP–OHP upon exposure to DI water. Black triangles indicate resistance of graphene sensor functionalized with only GBP upon exposure to S. aureus . Green stars indicate resistance of graphene sensor functionalized with GBP–OHP upon exposure to erythrocytes. Red circles indicate resistance of graphene sensor functionalized with GBP–OHP upon exposure to S. aureus . Dotted line indicates elution with DI water. Inset shows image of the flow-through measurement system. Scale bar is 1 cm. Concentration of the bacterial cells used for the assays is 10 6 CFU ml −1 , and the concentration of erythrocytes is 40% haematocrit. Full size image Activities of the immobilized GBP–OHP toward S. aureus , H. pylori , and erythrocytes were compared via fluorescent assays ( Fig. 3c–e , respectively). The concentrations of bacterial cells used for the assays were 10 6 colony-forming units (CFU) ml −1 and the concentration for erythrocytes was 40% haematocrit. The assays clearly show higher binding to bacterial cells, evident by the higher fluorescent density. The specificity of the interaction of S. aureus cells with GBP–OHP peptides was further analysed via flow-through electrical measurements of the graphene sensors ( Fig. 3f ). Following elution with deionized (DI) water, the response of GBP–OHP towards S. aureus is fourfold larger than the response of a GBP-functionalized sensor or a GBP–OHP sensor exposed to erythrocytes. Single bacterium detection Detection of bacteria at the single-cell level is a critical goal for biosensors due to the extremely low MID of many bacteria [18] , [33] , [40] . To investigate the responsiveness of the graphene nanosensors towards single bacterial cells, time-dependent resistance data and optical measurements were carried out in parallel. Importantly, as shown in Fig. 4a , simultaneous collection of electrical and fluorescence data from bare graphene sensors in the presence of fluorescently labelled E. coli cells clearly indicate a discrete change in electrical resistance corresponding to the binding and unbinding of a single bacterial cell from the graphene surface ( Supplementary Movie 1 ). The ∼ 0.6% decrease in resistance owing to binding of bacteria is readily explained by the fact that Gram-negative bacteria such as E. coli possess an outer membrane with negatively charged lipopolysaccharide, indicating p-type behaviour of the graphene transducer consistent with other studies [11] . 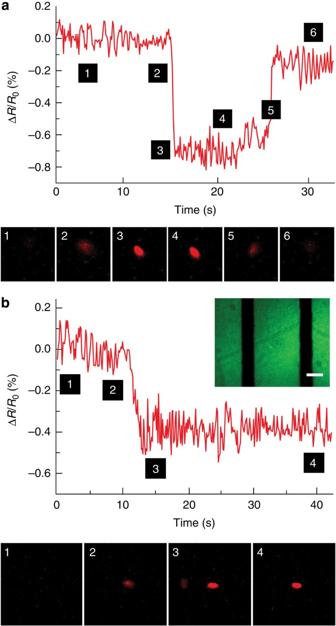Figure 4: Single-bacterium detection. (a) Electrical resistance (upper) and fluorescence (lower) data recorded simultaneously versus time showing binding/unbinding of a singleE. colibacterium on a bare graphene nanosensor. Images are (12 μm)2. (b) Resistance (upper) and optical (lower) data recorded simultaneously versus time showing binding of a singleE. colibacterium on a peptide-functionalized graphene nanosensor. Images are (20 μm)2. Inset shows fluorescent image of peptide-functionalized graphene surface (green), with the black regions representing electrodes. Scale bar is 250 μm. Figure 4: Single-bacterium detection. ( a ) Electrical resistance (upper) and fluorescence (lower) data recorded simultaneously versus time showing binding/unbinding of a single E. coli bacterium on a bare graphene nanosensor. Images are (12 μm) 2 . ( b ) Resistance (upper) and optical (lower) data recorded simultaneously versus time showing binding of a single E. coli bacterium on a peptide-functionalized graphene nanosensor. Images are (20 μm) 2 . Inset shows fluorescent image of peptide-functionalized graphene surface (green), with the black regions representing electrodes. Scale bar is 250 μm. Full size image Next, we determined the effect of the immobilized AMPs on bacterium binding. The inset of Fig. 4b shows a fluorescent image of the graphene nanosensor functionalized with fluorescein isothiocyanate-labelled GBP–OHP. The result suggests uniform coverage of the graphene surface with peptides and selective recognition of the peptide towards graphene relative to the gold electrodes. Simultaneous resistance and optical data were recorded on graphene sensors functionalized with GBP–OHP ( Fig. 4b ). Significantly, compared with the bare graphene nanosensor ( Fig. 4a ), peptide-coated electrodes display bacterium binding without concomitant unbinding ( Supplementary Movie 2 ), suggesting a strong interaction between the bacterium and immobilized peptides. Wireless remote query monitoring of S. aureus A major functionality of the sensor construction is the wireless remote query capability. Certain strains of S. aureus are notoriously antibiotic-resistant and responsible for over 500,000 post-surgical wound infections in the United States each year [41] , [42] . S. aureus has been reported to survive up to 9 weeks on standard plastic and similar dry hospital environments [42] . To simulate the use of graphene wireless sensors in hospital sanitation and biohazard monitoring, we interfaced the nanosensors with an intravenous (IV) bag ( Fig. 5a ). Sensor stability on the IV bag was tested against mechanical stress associated with bag crumpling by measuring the change in sheet resistance and transmittance of the graphene ( Supplementary Fig. S7 ). 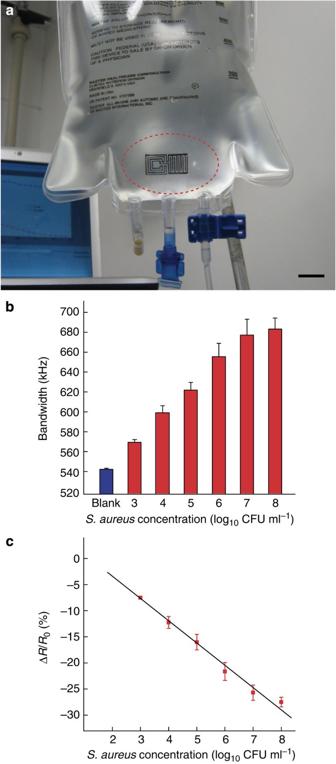Figure 5: Wireless monitoring ofS. aureus.(a) Optical image of the graphene wireless sensor integrated onto the surface of an IV bag. Scale bar is 1 cm. (b) Bandwidth of the sensor resonance corresponding to various concentrations ofS. aureuscells incubated on the sensor surface and dried. (c) Percentage change in graphene resistance versus concentration ofS. aureus. Error bars show s.d. (N=3). Figure 5: Wireless monitoring of S. aureus. ( a ) Optical image of the graphene wireless sensor integrated onto the surface of an IV bag. Scale bar is 1 cm. ( b ) Bandwidth of the sensor resonance corresponding to various concentrations of S. aureus cells incubated on the sensor surface and dried. ( c ) Percentage change in graphene resistance versus concentration of S. aureus . Error bars show s.d. ( N =3). Full size image Next, 1μl solutions containing various concentrations (10 3 –10 8 CFU ml −1 ) of bacterial cells were allowed to dry on the sensor surface for 30 min. The change in graphene resistance upon bacterial binding was wirelessly monitored as the bandwidth change in the sensor resonance curve [10] (Methods). Figure 5b plots the bandwidth of the sensor corresponding to different concentrations of S. aureus cells incubated on the sensor surface. The percentage change in graphene resistance is depicted in Fig. 5c ; significantly, detection limits of 1 bacterium μl −1 were achievable in wireless operation mode. Tooth platform monitoring of breath and saliva To investigate the performance of the sensor when directly integrated with biological tissue, the sensor was biotransferred onto the surface of a bovine tooth ( Fig. 6a ). Teeth are in constant contact with breath and saliva, which represent rich biologic media that can be probed for the presence of disease, infectious agents or metabolic changes [43] , [44] , [45] . Monitoring dynamic characteristics of respiration, including the presence of biomarkers and volatile organic compounds in exhaled breath, is of growing interest in non-invasive disease diagnosis [44] , [45] , [46] . Significantly, integration of the tooth sensor enabled remote monitoring of breath when exhaling on the tooth ( Supplementary Movie 3 ). 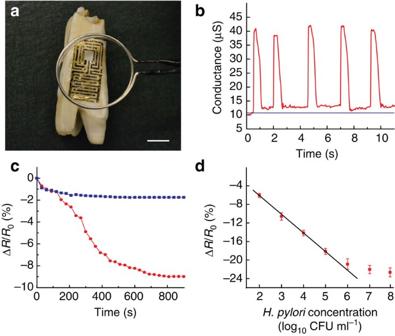Figure 6: Tooth sensor monitoring of breath and saliva. (a) Optical image of the graphene wireless sensor biotransferred onto the surface of a tooth. Scale bar is 1 cm. (b) Electrical conductance versus time upon exposure of the sensor to pulses of exhaled breath (red line). Baseline conductance is shown as blue line. (c) Percentage change in graphene resistance versus time following exposure to∼100H. pyloricells in human saliva (red line). The response to 'blank' saliva solution is shown as blue line. (d) Percentage change in graphene resistance versus concentration ofH. pyloricells. Error bars show s.d. (N=3). Figure 6b depicts the real-time change in graphene conductance on exposure to breath. Importantly, the sensor shows rapid response to breath, and the signal was observed to terminate quickly after the breath pulse. Figure 6: Tooth sensor monitoring of breath and saliva. ( a ) Optical image of the graphene wireless sensor biotransferred onto the surface of a tooth. Scale bar is 1 cm. ( b ) Electrical conductance versus time upon exposure of the sensor to pulses of exhaled breath (red line). Baseline conductance is shown as blue line. ( c ) Percentage change in graphene resistance versus time following exposure to ∼ 100 H. pylori cells in human saliva (red line). The response to 'blank' saliva solution is shown as blue line. ( d ) Percentage change in graphene resistance versus concentration of H. pylori cells. Error bars show s.d. ( N =3). Full size image Next, we explored the response of the tooth sensors to H. pylori , a Gram-negative pathogen found in the stomach and saliva, which is estimated to be responsible for the development of over 90% of duodenal ulcers and stomach cancers [47] , [48] . In particular, we investigated the ability of the graphene–AMP sensors to selectively recognize H. pylori cells in human saliva. Tooth sensors were first exposed to a solution of saliva and the signal was allowed to stabilize. Next, H. pylori cells dissolved in a pooled sample of saliva were allowed to come into contact with the tooth sensor. Optical experiments with fluorescently labelled bacterial cells verified that the immobilized AMPs recognize and bind bacterial cells, after incubating in saliva for ca. 15 min. Figure 6c depicts the real-time change in graphene resistance on exposure to a 1μl sample of human saliva containing ∼ 100 H. pylori cells, while 1 μl of 'blank' saliva solution without any bacterial cells was used as a control. Figure 6d thus depicts the percentage change in resistance as a function of bacterial concentration after 10 min by wirelessly recording the characteristic frequencies at resonance [25] , [49] , [50] (Methods). A linear relationship was observed between the logarithm of bacteria concentration and the resistance change up to a concentration of 10 6 bacterial cells, with a lower detection limit of ∼ 100 cells. Promisingly, this latter value is two orders of magnitude less than the MID for H. pylori [40] . This demonstrates the natural specificity possessed by AMPs in recognizing and binding to pathogenic bacterial cells, even in the presence of complex saliva interferrents such as epithelial cells, proteins and immunoglobulins. This work realizes the direct interfacing of highly sensitive and selective graphene nanosensors with natural biomaterials for single-cell detection, and for passive, wireless monitoring. The sensor is realized via the synergistic, hierarchical integration of a variety of smart material properties. The surface-dominated graphene sensing elements allow for intimate, robust conformability onto biological tissues or teeth. As a sensing system, the resulting device has several key meritorious properties, including extremely high sensitivity owing to the graphene network, biotransferability offered by the water-soluble silk fibroin platform, broadly selective biorecogniton enabled by robust AMPs and the ability to achieve battery-free, wireless remote query operation via the incorporation of a parallel resonant circuit with a gold thin-film-patterned meander line inductor [51] , [52] and interdigitated capacitive electrodes. Silk thin films serve as an ideal 'temporary tattoo' platform owing to their optical transparency, mechanical robustness, biotransferability, flexibility and biocompatibility [22] , [23] . When crystallized in air, the silk fibroin secondary structure kinetically favours silk I formation, a disordered collection of α-helices and random coils resulting in aqueous solubility. Such films possess programmable solubility rates dependent on β-sheet content and fibroin concentration, making them ideal substrates for the clean and controlled transfer of graphene to biological and material surfaces. Functionalization of graphene nanosensors with bifunctional peptides enables efficient recognition of pathogenic bacteria. Previous results showed that GBPs display high surface coverage and strong binding activity due to π-stacking interactions between aromatic residues [27] . Graphene sheets functionalized with OHP, an AMP isolated from the skin of the frog species Odorrana grahami , enabled broadband detection of Gram-positive and Gram-negative bacteria. Previous studies showed that bacterial binding of AMPs are observed as a precursor to bacteriocidal activity [32] , and OHP displays broad activity against: H. pylori , a Gram-negative species found in the stomach and saliva, which is responsible for ulcers and stomach cancers; E. coli , a Gram-negative species found in the lower intestine of endotherms with known strains capable of acute food poisoning and urinary tract infections resulting from unhygienic meat and dairy preparation; and S. aureus , a Gram-positive species found on skin flora and hospital equipment that is notoriously drug-resistant. OHP is also known to exert antimicrobial activity against methicillin-resistant strains of S. aureus [39] . A single-layer thin-film inductor–capacitor (LC) resonant circuit integrated in parallel with the resistive graphene monolayer enables wireless readout and battery-free operation. The change in conductance of the graphene nanosensor on binding of pathogenic bacteria is resolved from changes in the characteristic frequencies and bandwidth of sensor resonance. Both are quantities that are dominatingly determined by the resonant circuit, and readout can thus be insensitive to the mutual inductance (coupling coefficient) between the sensor and reader coil. Therefore, the relative alignment and location of the sensor with respect to the reader antenna is unimportant, and flexible operation is achieved. However, we note that improvements in sensor performance will require better control over potential non-uniformities in analyte coverage, and a reduction of artifacts such as air bubbles in the case of immersion in liquid. In conclusion, direct integration of highly sensitive graphene nanosensors with biomaterials such as tooth enamel has enabled battery-free sensors for remote monitoring of pathogenic bacteria. This work thus represents a fundamentally new paradigm in biochemical detection, and may provide an in situ , first-order monitoring and detection system for applications including point-of-care diagnostics, hospital sanitation monitoring and food safety analysis. Yet, these results are only a prototype, 'first generation' platform for interfaced graphene nanosensors. Owing to the semiselective nature of the interaction of AMPs with pathogenic bacteria, differentiation of multiple species of pathogenic bacteria has not been achieved. Future work will involve exploring strategies to improve this selectivity via investigations into multi-ligand [53] , [54] and aptamer-based capture agents [26] , [55] , and antibody-based biorecognition molecules with improved stability [56] to provide stringent discrimination between species of pathogenic bacteria. Alternative strategies for covalent and non-covalent functionalization of graphene sensors will also be explored [57] . Finally, future challenges in the sensor development will involve further miniaturization of the wireless coil for integration onto a smaller footprint (such as a human tooth) [58] , [59] and testing of the platform on in vivo systems, including tissue and teeth in living animals and humans. Reagents and biological agents The bifunctional peptide GBP–OHP (HSSYWYAFNNKT-GGGGLLRASSVWGRKYYVDLAGCAKA) containing a graphene-binding motif linked to the AMP OHP via a triglycine linker were chemically synthesized and obtained from Peptide 2.0 Inc (Chantilly, VA, USA). Heat-killed pathogenic Gram-negative bacterial cells of E. coli O157:H7 and H. pylori were purchased from KPL (Gaithersburg, MD, USA). Heat-killed Gram-positive bacterial cells of S. aureus were purchased from Invitrogen Inc. The human saliva sample was purchased from Lee Biosolutions (St Louis, MO, USA). The stock solution of peptide was prepared by reconstitution of the lyophilized powder in DI water. Different concentrations of bacterial samples were prepared from stock solutions via dilution in DI water or human saliva. Phosphate-buffered saline (PBS) consisting of 137 mM NaCl, 2.7 mM KCl, 4.4 mM Na 2 HPO 4 and 1.4 mM KH 2 PO 4 (pH 7.4), FeCl 3 , sodium carbonate and lithium bromide for the processing of silk were purchased from Sigma Aldrich (St Louis, MO, USA). Preparation of silk films Bombyx mori cocoons were boiled in 0.02 M Na 2 CO 3 for 30 min followed by thorough rinsing with water. The degummed silk was then dissolved in 9.3M aqueous lithium bromide and the solution was dialyzed to remove excess salt. The resulting aqueous solutions were 6–10% (w/v) fibroin and were preserved by storage at 5 °C. Silk films were made by casting fibroin solutions onto polydimethylsiloxane (PDMS) and drying in air for 12–24 h, depending on the thickness. When crystallized in air, silk fibroin secondary structure kinetically favours silk I formation and ca. 50μm thick films. For the preparation of fluorescent silk films for silk dissolution test, silk fibroin solution was mixed with fluorescence dye and allowed to crystallize overnight. Fabrication of graphene/silk sensors Chemical vapour deposition-grown graphene monolayers from Ni thin films were released and transferred onto PDMS stamps by removal of the Ni layer in FeCl 3 . Graphene was then transfer printed onto the silk films. Clean transfer of graphene onto silk was achieved via moistening of the silk surface using a wet cotton swab. Planar inductive and capacitive elements were then incorporated onto the graphene/silk samples to enable wireless interrogation. A meander line design for the inductive element was deposited on the graphene nanosensor via shadow mask-assisted electron beam evaporation of gold (150–200 nm). Biotransfer onto biomaterials Integration of the sensor onto biomaterial surfaces was achieved via dissolution of the supporting silk substrate. In the case of dry surfaces such as a tooth, a moistened cotton swab was used to slightly wet the surface. The graphene–Au electrode sensing elements on the temporary silk films were then carefully aligned and placed on the tooth surface with the device side facing down. The temporary silk film platform was gradually dissolved off by application of water, leaving the ultra-thin sensors intimately attached to the surface by van der Waals forces. In the case of wet surfaces such as muscle tissue, dissolution of the silk film was faster. IV bags (Baxter ViaFlex) used for the study were provided by the Princeton University Medical Center. Graphene functionalization with AMPs The bifunctional peptide GBP–OHP was dissolved in DI water at a concentration of 1 mg ml −1 . A volume of 5 μl of the peptide solution was dropped onto the graphene and incubated for 15 min, followed by washing with DI water and drying. Single-bacterium detection measurements Electrical measurements for the detection of a single bacterium were performed with a lock-in detection system using the Stanford Research Systems 810 DSP lock-in amplifier. A signal of 50 mV was used with a modulation frequency of 30–70 Hz with zero DC bias to avoid electrochemical reactions. The resistance of the graphene sensor was monitored continuously in the presence of analyte samples of various dilutions of bacterial cells. Bacterial cells for optical monitoring and for AMP–bacteria-binding density studies were fluorescently labelled with propidium iodide (PI) in a manner similar to previous studies [30] . Stock solutions of PI, nucleic acid stain (Molecular Probes, Eugene, OR, USA), were made from solid form by dissolving PI (molecular weight=668.4) in DI water at 1 mg ml −1 (1.5 mM) and stored at 4 °C, protected from light. Heat-killed bacterial cells rehydrated in PBS were then incubated with 3 μM solution of PI (made by diluting the 1 mg ml −1 stock solution 1:500 in buffer) for 10–15 min. After incubation, the cells were pelleted by centrifugation and removal of the supernatant, and were resuspended in DI water or 1×PBS buffer. The binding pattern of the different bacterial cells was imaged using a Zeiss Axiovert inverted microscope and recorded with a Zeiss AxioCam digital camera. For real-time detection of bacterial cells ( E. coli O157: H7), a 1 μl sample containing 100 bacterial cells was pipetted onto the graphene sensors. Simultaneous bright field and fluorescent data were recorded together with lock-in resistance data, with the focal plane set on the graphene surface to identify the events when the bacterial cells came close to the sensor. The motion of the bacterial cells was tracked with the help of video spot tracker, a custom automated tracking software (freely available at http://cismm.org/downloads/ ), and the manual tracking plugin of the National Institutes of Health's ImageJ software. Wireless sensing experiments A single-layer LC resonant circuit, integrated in parallel with the resistive (R) graphene monolayer, formed the basis of the wireless readout unit. The reader device consisted of a two-turn coil antenna connected to a frequency response analyzer (HP 4191A RF impedance analyzer). The wireless reader, which was powered by an alternating current source, was responsible for wirelessly transmitting power and receiving sensor data from the remote passive sensor, all via inductive coupling ( Supplementary Fig. S8 ). Passing an AC signal through the antenna generated a magnetic field, inducing current via mutual inductance in the coil of the sensing element (Faraday's law), and finally resulting in a potential drop that depended on the conductance of the graphene nanosensor. Any change in the conductivity of the sensor system—resulting from biological or chemical changes occurring at the transducer surface—was reflected as a change in the frequency characteristics (namely bandwidth) around the resonance point [25] , [49] , [60] . This allowed the reader to wirelessly interrogate the sensing element by measuring the complex impedance of the system. The change in the capacitance ( C ) of the graphene-interdigitated electrode sensing system was deduced from the resonance frequency shift ( f ), the expression for which is The bandwidth of the sensor's resonant network ( B ) was measured from the magnitude of the sensor impedance ( Supplementary Fig. S9 ) and used to calculate the change in resistance ( R ) of the graphene–electrode sensing element on binding of the bacterial cells. The expression for the change in resistance of the system is Frequency measurements on the sensor system were performed by monitoring the complex impedance spectrum of the system ( Supplementary Fig. S10 ). The frequency at which the imaginary part of the sensor impedance vanishes ( f z ) was continually monitored and used to calculate the graphene resistance: where, L is the inductance of the system and can be measured separately. The equivalent circuit of the sensing element was used to calculate the bandwidth of the reader-sensor system, and the input impedance of the system was viewed by the reader device ( Supplementary Fig. S11 and Supplementary Methods ). How to cite this article: Mannoor, M.S. et al . Graphene-based wireless bacteria detection on tooth enamel. Nat. Commun. 3:763 doi: 10.1038/ncomms1767 (2012).